Gene regulation and priming by topoisomerase IIα in embryonic stem cells Topoisomerases resolve torsional stress, while their function in gene regulation, especially during cellular differentiation, remains unknown. Here we find that the expression of topo II isoforms, topoisomerase IIα and topoisomerase IIβ, is the characteristic of dividing and postmitotic tissues, respectively. In embryonic stem cells, topoisomerase IIα preferentially occupies active gene promoters. Topoisomerase IIα inhibition compromises genomic integrity, which results in epigenetic changes, altered kinetics of RNA Pol II at target promoters and misregulated gene expression. Common targets of topoisomerase IIα and topoisomerase IIβ are housekeeping genes, while unique targets are involved in proliferation/pluripotency and neurogenesis, respectively. Topoisomerase IIα targets exhibiting bivalent chromatin resolve upon differentiation, concomitant with their activation and occupancy by topoisomerase IIβ, features further observed for long genes. These long silent genes display accessible chromatin in embryonic stem cells that relies on topoisomerase IIα activity. These findings suggest that topoisomerase IIα not only contributes to stem-cell transcriptome regulation but also primes developmental genes for subsequent activation upon differentiation. DNA topoisomerases are among the most conserved proteins [1] , [2] , [3] explained by their key function in relieving torsional stress of DNA during fundamental cellular processes such as replication, transcription, recombination, chromatin remodelling, chromosome condensation and segregation [4] , [5] , [6] . Mammals have two classes of topoisomerases: Type I, that pass one strand of DNA through a break in the opposing strand and type II, that pass a region of duplex from the same or a different molecule through a double-stranded gap generated in the DNA [1] , [4] , [5] , [6] . Mammalian cells encode two type II isozymes, topoisomerase II α (TOP2α) and β (TOP2β), that have highly identical N-terminal ATPase and central core domains [7] , [8] . However, they differ in their C-termini as well as expression patterns and cannot compensate for each other in vivo [8] , [9] , [10] . Genetic deletion of TOP2β uncovered its critical role in neuronal development [11] , while TOP2α inactivation is embryonic lethal [8] , [12] . TOP2β is highly expressed in terminally differentiated cells including postmitotic neurons [13] , [14] , [15] , whereas TOP2α is very abundant in rapidly dividing cells, such as pluripotent embryonic stem cells (ESCs) [16] , [17] , [18] . We had previously shown that induction of stem-cell differentiation towards neuronal lineage accompanies a switch in the expression from TOP2α to TOP2β [16] . Given this switch in expression of the two topo II isozymes when cells transit from actively dividing, pluripotent state to a postmitotic, terminally differentiated state, we were tempted to investigate the stem cell-specific function of TOP2α as well as similarities and differences in targets with TOP2β. Furthermore, given a plethora of factors that are being implicated in the regulation of stem cell pluripotency and differentiation [19] , [20] , [21] , [22] , [23] , [24] , we were interested to uncover how these crucial enzymes contribute to this process. Here we attempt to unravel topoisomerase II targets and function in highly proliferating, pluripotent stem cells and its similarities and differences with postmitotic, terminally differentiated cells. We address this by employing an established murine neuronal differentiation system that progresses through defined stages with high synchrony and homogeneity that closely resemble in vivo characteristics [25] , [26] , [27] . We show that in pluripotent stem cells, TOP2α preferentially binds to promoter regions that are marked with the active histone mark H3K4me2 and largely transcribed. Interestingly, a target comparison of the two topo II isoforms in proliferating stem cells and postmitotic neurons revealed that although common targets are involved in housekeeping function, TOP2α-specific targets are associated with proliferation and stem cell program and TOP2β-specific targets are enriched for cell-fate commitment and neurogenesis. A subset of TOP2α targets that are not expressed in ES cells are developmental genes and exhibit bivalent chromatin marks. Induction of differentiation accompanies resolution of bivalent marks at these promoters that parallels their transcriptional induction and occupancy by TOP2β. Similar dynamics in binding of Topo II isoforms and target gene expression is also observed for genes in the largest length class. TOP2α activity keeps these long silent genes in an accessible chromatin state in ESCs, possibly as a prerequisite for later activation. Furthermore, catalytic inhibition of TOP2α in ESCs results in changes in chromatin state and altered RNA Pol II kinetics at target promoters that accompanies misregulated gene expression. Taken together, our data provide strong evidence for a gene regulatory role for TOP2α as well as an isozyme-specific function at a distinct set of targets in the context of cellular differentiation. Expression of topo II isoforms defines developmental state A number of previous studies including our work revealed a switch in the expression from TOP2α to TOP2β during neuronal differentiation [13] , [15] , [16] . We next attempted to characterize whether the expression switch of topo II isoforms is a general feature of postmitotic tissues. Using publically available mouse RNA-Seq data sets, we found that dividing cells show higher expression of Top2a , while fully differentiated tissues from all three lineages exclusively express Top2b ( Fig. 1a,b ). To substantiate our findings, we analysed previously published transcriptome data from various stages of embryonic cortical neurogenesis where rapidly dividing neuronal progenitor cells in the ventricular zone progress through an intermediate stage in the subventricular zone to generate postmitotic, mature neurons in the cortical plate [28] . These data clearly showed a switch from Top2a to Top2b during cortical neurogenesis ( Fig. 1c ). Moreover, the same switch was further appreciated during in vitro differentiation of ESCs into neurons ( Fig. 1d ). This led us to conclude that Top2a and Top2b expression are characteristics of dividing, pluripotent and postmitotic, differentiated tissues, respectively, and this transition in expression is a universal feature across all lineages during development. 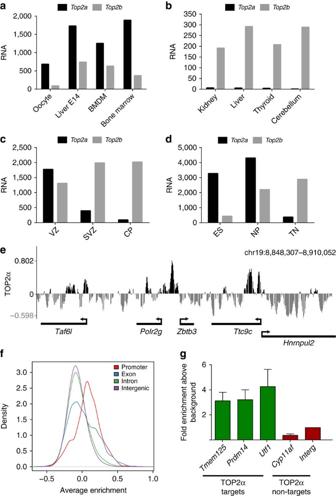Figure 1: Switch in the expression of Topo II isoforms marks developmental transition. (a) Publically available RNA-Seq data sets were analysed to investigate the expression pattern ofTop2aandTop2bin different tissues. Bar plots show the expression levels ofTop2aandTop2bin rapidly dividing tissues. RNA represents normalized tag counts from at least two biological replicates. These RNA-Seq data sets were normalized and analysed together to minimize library size variations on expression levels (BMDM=bone marrow derived macrophages). (b) Bar plots showing the expression levels ofTop2aandTop2bin fully differentiated tissues derived from 8-week-old adult mice. (c) Bar plots showing expression levels ofTop2aandTop2bduring cortical neurogenesis (VZ, ventricular zone; SVZ, subventricular zone; CP, cortical plate). (d) Bar plots showing expression levels ofTop2aandTop2bduring stem cell differentiation to neurons (ESC, embryonic stem cells; NP, neuronal progenitors; TN, terminally differentiated neurons). (e) Genome browser screen shot from a segment of chromosome 19 giving an example of localization patterns of TOP2α in ESCs. Theyaxis represents log2 enrichments (IP/input). (f) Distribution of TOP2α enrichments in different genomic regions. The fully tiled chromosome 19 was hierarchically divided into promoter, exon, intron and intergenic regions and for each region TOP2α enrichments were calculated by averaging over all probes that mapped to the particular genomic class. (g) ChIP-qPCR for TOP2α enrichment at a few target gene promoters and non-target sites in ESCs. Average enrichments, from three separate assays, are plotted on theyaxis as the ratio of precipitated DNA (bound) to the total input DNA and further normalized to a control region Interg (Intergenic region). Error bars indicate s.e.m. Figure 1: Switch in the expression of Topo II isoforms marks developmental transition. ( a ) Publically available RNA-Seq data sets were analysed to investigate the expression pattern of Top2a and Top2b in different tissues. Bar plots show the expression levels of Top2a and Top2b in rapidly dividing tissues. RNA represents normalized tag counts from at least two biological replicates. These RNA-Seq data sets were normalized and analysed together to minimize library size variations on expression levels (BMDM=bone marrow derived macrophages). ( b ) Bar plots showing the expression levels of Top2a and Top2b in fully differentiated tissues derived from 8-week-old adult mice. ( c ) Bar plots showing expression levels of Top2a and Top2b during cortical neurogenesis (VZ, ventricular zone; SVZ, subventricular zone; CP, cortical plate). ( d ) Bar plots showing expression levels of Top2a and Top2b during stem cell differentiation to neurons (ESC, embryonic stem cells; NP, neuronal progenitors; TN, terminally differentiated neurons). ( e ) Genome browser screen shot from a segment of chromosome 19 giving an example of localization patterns of TOP2α in ESCs. The y axis represents log2 enrichments (IP/input). ( f ) Distribution of TOP2α enrichments in different genomic regions. The fully tiled chromosome 19 was hierarchically divided into promoter, exon, intron and intergenic regions and for each region TOP2α enrichments were calculated by averaging over all probes that mapped to the particular genomic class. ( g ) ChIP-qPCR for TOP2α enrichment at a few target gene promoters and non-target sites in ESCs. Average enrichments, from three separate assays, are plotted on the y axis as the ratio of precipitated DNA (bound) to the total input DNA and further normalized to a control region Interg (Intergenic region). Error bars indicate s.e.m. Full size image TOP2α preferentially binds gene promoters To get insights into the embryonic stem cell-specific function of TOP2α, we performed chromatin immunoprecipitation for TOP2α in mouse ESCs and investigated its genomic binding patterns using the array platform previously described [16] . Visual inspection of genomic regions suggested targeting of TOP2α to distinct genomic sites including promoters ( Fig. 1e ). A comprehensive and unbiased analysis of TOP2α enrichment along chromosome 19 revealed a preferential enrichment for TOP2α at promoters, slight enrichment at exons and none at introns and intergenic regions ( Fig. 1f ). These observations were validated by independent ChIP-qPCRs ( Fig. 1g ). Such targeting of TOP2α to gene promoters prompted us to investigate its possible role in transcriptional regulation in ESCs. TOP2α targets exhibit open chromatin and are transcribed To shed light into the relationship of TOP2α binding with certain key histone modifications and expression state of target genes, we analysed our existing ChIP-Seq data sets for H3K4me2, H3K27me3 and RNA Pol II as well as RNA-Seq data from ESCs [16] and compared this with TOP2α occupancy. Visual inspection revealed various combinations in which chromatin marks occurred at TOP2α targets and associated with transcription state of genes ( Fig. 2a ). To gain global insights into these patterns, we performed genome-wide correlation analysis at promoters that revealed a strong correlation of TOP2α binding with the active histone mark H3K4me2 ( R 2 : 0.67), RNA Pol II occupancy ( R 2 : 0.48) and active transcription ( R 2 : 0.46) but a weak correlation with the repressive mark H3K27me3 ( R 2 : 0.23) ( Fig. 2b and Supplementary Fig. S1a ). These regions are further not enriched for other repressive histone modifications, supporting the strong association of TOP2α with active chromatin ( Supplementary Fig. S1c ) [29] , [30] . Correlation of TOP2α with H3K4me2 was also observed at other genomic regions, however, driven by lower enrichments ( Supplementary Fig. S1b ). Heat map visualization at promoters supported these observations revealing that the majority of TOP2α-bound genes display H3K4me2 mark and a significant fraction of these genes are Pol II bound and actively transcribed ( Fig. 2c , class I and II). Moreover, genes that were not bound by TOP2α showed an overall lower H3K4me2 enrichment, expression and Pol II binding ( Fig. 2c , class IV). Taken together, these data clearly show that the majority of TOP2α-bound genes are expressed in ESCs and are defined by an active chromatin state. 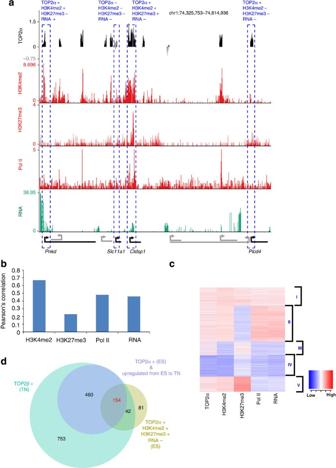Figure 2: TOP2αtargets are defined by an active chromatin state and are largely transcribed. (a) UCSC genome browser screen shot from a 290-kb region on chromosome 1 displaying enrichments of TOP2α, H3K4me2, H3K27me3 and Pol II occupancy (four upper panels) and RNA (FPKM values from RNA-Seq) (lowermost panel). Genes are depicted below with arrows indicating direction of transcription. (b) Histogram showing Pearson’s correlation of TOP2α occupancy with H3K4me2, H3K27me3, Pol II binding and mRNA expression at all promoters. (c) Heat map depicting TOP2α, H3K4me2, H3K27me3 and Pol II enrichment and corresponding mRNA expression levels at each promoter. Promoters were clustered (shown by roman numerals) usingk-means clustering with k=5. Each row represents one promoter, red: high enrichment/expression, blue: low enrichment/expression. (d) Venn diagram illustrating the overlap of TOP2α target genes that are not expressed in ESCs, display bivalent histone marks with genes that become occupied by TOP2β and genes that are upregulated in TN. Figure 2: TOP2 α targets are defined by an active chromatin state and are largely transcribed. ( a ) UCSC genome browser screen shot from a 290-kb region on chromosome 1 displaying enrichments of TOP2α, H3K4me2, H3K27me3 and Pol II occupancy (four upper panels) and RNA (FPKM values from RNA-Seq) (lowermost panel). Genes are depicted below with arrows indicating direction of transcription. ( b ) Histogram showing Pearson’s correlation of TOP2α occupancy with H3K4me2, H3K27me3, Pol II binding and mRNA expression at all promoters. ( c ) Heat map depicting TOP2α, H3K4me2, H3K27me3 and Pol II enrichment and corresponding mRNA expression levels at each promoter. Promoters were clustered (shown by roman numerals) using k -means clustering with k=5. Each row represents one promoter, red: high enrichment/expression, blue: low enrichment/expression. ( d ) Venn diagram illustrating the overlap of TOP2α target genes that are not expressed in ESCs, display bivalent histone marks with genes that become occupied by TOP2β and genes that are upregulated in TN. Full size image Cooperativity of Topo II isoforms at developmental genes We further observed a class of TOP2α target genes ( n =277) that were marked with H3K4me2 as well as H3K27me3 and not RNA Pol II enriched or transcribed in ESCs (cluster V in Fig. 2c , Supplementary Fig. S2a ). This suggested that TOP2α is recruited to bivalent promoters in the absence of Pol II. Interestingly, a majority of these genes (71%, n =196) were targeted by TOP2β in terminally differentiated neurons ( Fig. 2d ), that paralleled resolution of bivalent mark concomitant with their expression (79%, n =154 out of 196) ( Fig. 2d , Supplementary Fig. S2b ). GO term analysis for these genes revealed enrichment for developmental processes such as cell-fate commitment, tissue development and cell signalling ( Supplementary Table S1 ). These data suggested a possible role of TOP2α in concert with the surrounding chromatin to mark differentiation genes for later activation. Topo II targets mark cell-type and housekeeping function As previously identified target genes of TOP2β uncovered its function in regulating neuronal identity [16] , we next investigated similarities and differences between target genes of TOP2α and TOP2β in proliferating stem cells and postmitotic neurons, respectively. Interestingly, approximately half of the TOP2α-bound genes in stem cells become bound by TOP2β in postmitotic neurons ( Fig. 3a ). The TOP2α-unique target genes in ESCs are involved in signalling pathways and biosynthesis processes, while TOP2β-unique bound genes in neurons function in neurogenesis. However, the common topo II targets are involved in transcriptional regulation ( Fig. 3a ). 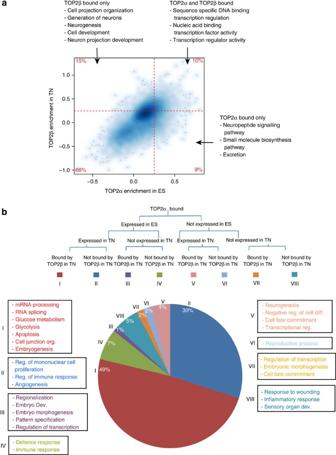Figure 3: TOP2αand TOP2β bind to common and distinct set of genes. (a) Scatter plot correlating the distribution of TOP2α enrichment in ES cells (xaxis) and TOP2β enrichment in postmitotic neurons (yaxis) on a genome-wide scale; each dot represents a single promoter. An arbitrary cutoff of 0.25 was set to identify common and unique targets for TOP2α and TOP2β in ES and TN cells, respectively. Significant GO enrichment terms are displayed for the three categories (only TOP2β-bound, commonly bound by TOP2α and TOP2β and only TOP2α-bound) within the corresponding quadrant. (b) Pie chart showing the distribution and GO enrichment terms of all TOP2α target genes categorized in eight classes depending on their expression state in ES cells and postmitotic neurons and based on their occupancy by TOP2β in terminal neurons (refer to the colour code and numbering with roman numerals in the figure). GO enrichment analysis was performed with DAVID functional classification tool and GO enriched categories are mentioned in boxes around the pie chart with corresponding roman numerals. Figure 3: TOP2 α and TOP2β bind to common and distinct set of genes. ( a ) Scatter plot correlating the distribution of TOP2α enrichment in ES cells ( x axis) and TOP2β enrichment in postmitotic neurons ( y axis) on a genome-wide scale; each dot represents a single promoter. An arbitrary cutoff of 0.25 was set to identify common and unique targets for TOP2α and TOP2β in ES and TN cells, respectively. Significant GO enrichment terms are displayed for the three categories (only TOP2β-bound, commonly bound by TOP2α and TOP2β and only TOP2α-bound) within the corresponding quadrant. ( b ) Pie chart showing the distribution and GO enrichment terms of all TOP2α target genes categorized in eight classes depending on their expression state in ES cells and postmitotic neurons and based on their occupancy by TOP2β in terminal neurons (refer to the colour code and numbering with roman numerals in the figure). GO enrichment analysis was performed with DAVID functional classification tool and GO enriched categories are mentioned in boxes around the pie chart with corresponding roman numerals. Full size image To uncover TOP2α function in pluripotent stem cells we performed a comprehensive analysis of all TOP2α-bound genes in relation to target gene transcription. Towards this, we defined eight classes of TOP2α target genes depending on their expression in ESCs and neurons and TOP2β binding in neurons ( Fig. 3b ). In line with strong correlation of TOP2α binding with RNA Pol II and H3K4me2 enrichment, we found that almost 90% of TOP2α-bound genes in ESCs are expressed. Furthermore, 49% of TOP2α target genes that show housekeeping function stay expressed and become bound by TOP2β in postmitotic neurons ( Fig. 3b ). Seven per cent of TOP2α-bound genes are specifically expressed in ESCs and are not bound by TOP2β in postmitotic neurons. These genes are enriched for defense and immune response as reflected by many cytokine-related genes. These small molecules are known to contribute to ESC-specific features including maintenance of self-renewal [31] . Furthermore, 4% of TOP2α target genes that are not expressed in ESCs but become transcriptionally active and occupied by TOP2β in terminal neurons are involved in cell-fate commitment and neurogenesis. In summary, expressed genes exclusively targeted by TOP2α or TOP2β constitute cell type-specific transcription programs, while common targets are enriched for housekeeping function. TOP2α primes long silent genes for later activation Our data suggested that binding of TOP2α to genes that are not expressed in ESCs might pave the way for subsequent TOP2β binding and expression upon differentiation ( Figs 2d and 3b ). To investigate whether any sequence feature defines TOP2α-bound genes, we binned all TOP2α target genes into gene lengths of varying sizes and discovered that long genes (>250 kb) were mostly silent in ES cells but became expressed in neurons ( Fig. 4a ). These genes showed similar transcriptional dynamics during corticogenesis ( Fig. 4b ), further supporting our observations. Interestingly, these genes also become TOP2β targets in neurons ( Fig. 4c ). Considering the overall gene length distribution in the mouse genome the number of long genes being pre-bound by TOP2α in ESCs is substantial ( Supplementary Fig. S3a ). The majority of TOP2α-bound genes are between 1.5 and 125 kb of length, which resembles overall gene length distribution in the mouse genome ( Supplementary Fig. S3a ). Moreover, very similar fraction of genes from various length classes are expressed in both pluripotent and differentiated states ( Fig. 4a ). Importantly, however, genes longer than 125 kb significantly differ in their expression levels when comparing ESCs with terminally differentiated neurons. Only 30% of these TOP2α-bound genes (>250 kb) are expressed in pluripotent ESCs but all become expressed ( Fig. 4a ) and bound by TOP2β ( Fig. 4c ) in postmitotic neurons. Interestingly, about 50% of these genes (>250 kb) show bivalent chromatin, in agreement with their potential for expression upon differentiation ( Supplementary Fig. S3b ). GO term analysis of long length genes (>250 kb) revealed enrichment for neurogenesis-related genes ( Supplementary Table S2 ). As these silent genes become transcribed upon differentiation, we speculated whether they utilize TOP2α activity to acquire an accessible chromatin in ESCs in preparation for later activation. Towards this, we treated ESCs with ICRF-193 (ref. 32 ), an established TOP2α inhibitor ( Supplementary Fig. S4a,b ) and carried out FAIRE assay [33] , [34] in DMSO and ICRF-193-treated cells followed by next generation sequencing (FAIRE-Seq). Computational analysis revealed that inhibition of TOP2α activity in ESCs results in overall reduction in chromatin accessibility of the long silent genes, but not of other TOP2α targets ( Fig. 4d , Supplementary Fig. S3c ). These data collectively suggest a role for TOP2α in keeping long silent genes in an accessible chromatin state in ESCs before activation by TOP2β upon differentiation. 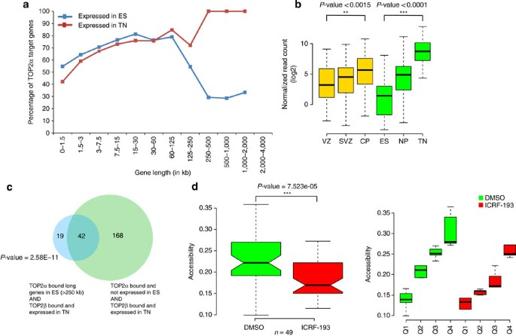Figure 4: TOP2αoccupancy in ES cells might prime long genes for later activation. (a) The distribution of percentage of genes expressed in ESCs and TNs. Thexaxis represents bins of gene length, whileyaxis represents percentage of TOP2α target genes expressed in each bin in ESCs (blue line) or TNs (red line). (b) Distribution of transcription differences for genes in the long length class (>250 kb) between various stages of corticogenesis (VZ, SVZ and CP; yellow) as well as stem cell differentiation to neurons (ES, NP and TN; green) as derived from RNA-Seq data. The box plots illustrate preferential expression of these genes upon terminal neuronal differentiation (VZ to CP;P-value <0.0015 (two asterisks) and ES to TN;P-value <0.0001 (three asterisks). Thexaxis depicts different cell types, whileyaxis represents normalized tag counts (log2 scale) from RNA-Seq data. Horizontal lines represent median, boxes represent 50% of data and whiskers represent 25% data on each side.P-values were calculated using paired Wilcoxon test from five replicates each of VZ, SVZ and CP and two replicates each of ES, NP and TN for the set of 61 genes. (c) Venn diagram illustrating a significant overlap of TOP2α-bound genes with length >250 kb with the class of genes that is TOP2α-bound in ESCs but is transcriptionally silent and becomes bound by TOP2β in TNs and transcribed.P-value was calculated using hypergeometric distribution. (d) FAIRE-Seq assay following ICRF-193 treatment reveals a significantly reduced chromatin accessibility at long silent genes (P-value=7.523e−05) (left panel). For this analysis, all peaks falling between TSS (including 1 kb upstream) and TTS (transcription termination site) for 49 genes (out of 61 for which enrichment was above input) were collated together and their median was assigned to each gene. Thexaxis indicates DMSO and ICRF-193 treatment conditions andyaxis represents chromatin accessibility as measured by FAIRE-Seq data.P-values were calculated using paired Wilcoxon test using two replicates. To further illustrate that these differences are not arising from any particular enrichment category of peaks, we divided the accessibility enrichment values in four equal bins (quartiles: Q1–Q4) (right panel). Box plots are plotted as mentioned in (b). Figure 4: TOP2 α occupancy in ES cells might prime long genes for later activation. ( a ) The distribution of percentage of genes expressed in ESCs and TNs. The x axis represents bins of gene length, while y axis represents percentage of TOP2α target genes expressed in each bin in ESCs (blue line) or TNs (red line). ( b ) Distribution of transcription differences for genes in the long length class (>250 kb) between various stages of corticogenesis (VZ, SVZ and CP; yellow) as well as stem cell differentiation to neurons (ES, NP and TN; green) as derived from RNA-Seq data. The box plots illustrate preferential expression of these genes upon terminal neuronal differentiation (VZ to CP; P -value <0.0015 (two asterisks) and ES to TN; P -value <0.0001 (three asterisks). The x axis depicts different cell types, while y axis represents normalized tag counts (log2 scale) from RNA-Seq data. Horizontal lines represent median, boxes represent 50% of data and whiskers represent 25% data on each side. P -values were calculated using paired Wilcoxon test from five replicates each of VZ, SVZ and CP and two replicates each of ES, NP and TN for the set of 61 genes. ( c ) Venn diagram illustrating a significant overlap of TOP2α-bound genes with length >250 kb with the class of genes that is TOP2α-bound in ESCs but is transcriptionally silent and becomes bound by TOP2β in TNs and transcribed. P -value was calculated using hypergeometric distribution. ( d ) FAIRE-Seq assay following ICRF-193 treatment reveals a significantly reduced chromatin accessibility at long silent genes ( P -value=7.523e−05) (left panel). For this analysis, all peaks falling between TSS (including 1 kb upstream) and TTS (transcription termination site) for 49 genes (out of 61 for which enrichment was above input) were collated together and their median was assigned to each gene. The x axis indicates DMSO and ICRF-193 treatment conditions and y axis represents chromatin accessibility as measured by FAIRE-Seq data. P -values were calculated using paired Wilcoxon test using two replicates. To further illustrate that these differences are not arising from any particular enrichment category of peaks, we divided the accessibility enrichment values in four equal bins (quartiles: Q1–Q4) (right panel). Box plots are plotted as mentioned in ( b ). Full size image TOP2α regulates ESC transcriptome We next attempted to ask whether enzymatic activity of TOP2α contributes to the transcriptional state of its target genes. Towards this, we performed genome-wide transcriptome profiling in ESCs treated with DMSO and ICRF-193 that revealed significant transcriptome changes following such TOP2α inhibition ( Fig. 5a ). Furthermore, most significantly up- and downregulated genes were direct TOP2α targets ( Fig. 5b,c ). For further analysis, we selected genes showing significant expression changes upon ICRF-193 treatment and focused on genes with high TOP2α enrichment ( Fig. 5c , exploded section). In this subset, GO term analysis of the downregulated genes revealed association with processes like metabolism, signalling, proliferation and transcriptional regulation ( Supplementary Table S3 ). Significantly upregulated genes were enriched in pathways related to cell-fate commitment, development and neurogenesis ( Supplementary Table S3 ). Moreover, the effect on cell-fate commitment genes could possibly not be driven by altered expression of TOP2α target metabolic genes, as the later constitutes only a small fraction of genes that change in expression upon ICRF-193 treatment ( Supplementary Fig. S5a ). Given that these metabolic genes show relatively high expression, TOP2α inhibitor may not be able to drastically alter their expression under low dose and short-treatment conditions ( Supplementary Fig. S5b ). We speculated if these misregulated genes rely on TOP2α for their transcriptional state, the observed expression changes should also be recapitulated during neuronal differentiation of stem cells when TOP2α is naturally shut down ( Fig. 1d ). We found majority of genes significantly downregulated after ICRF-193 treatment also display transcriptional silencing upon ESC differentiation into neurons ( Fig. 5d , Supplementary Table S4 ). These genes include players important for stem cell properties such as Eras and Fgf4 (refs 35 , 36 ). Furthermore, approximately half of the genes upregulated upon ICRF-193 treatment are also induced following neuronal differentiation and include genes known to be crucial for neuronal development like Chl1 and Mab21l2 (refs 37 , 38 ) ( Fig. 5e , Supplementary Table S5 ). These findings suggest a direct role for TOP2α enzymatic activity in regulating target gene expression, thereby defining ESC transcriptome. 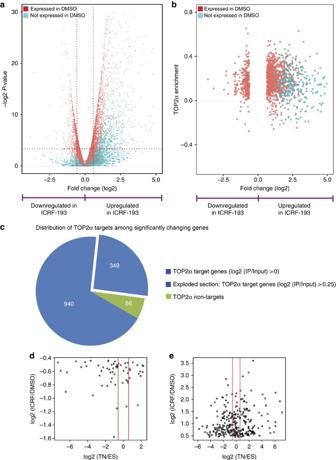Figure 5: Catalytic inhibition of TOP2αmisregulates target gene expression. (a) Volcano plot showing differentially expressed genes following ICRF-193 treatment as compared with DMSO in ESCs. Thexaxis shows fold changes in expression (log2 scale) and theyaxis refers to the associatedP-value (−log2 scale). The dotted red lines indicate the used cutoffs. Genes not expressed and expressed in DMSO treated samples are depicted in cyan and red respectively. (b) Scatter plot showing TOP2α enrichment at promoters (yaxis) of genes significantly misregulated (log2 scale) following ICRF-193 treatment (xaxis). (c) Pie chart representing the distribution of genes showing any TOP2α enrichment (log2 IP/input>0) or TOP2α enrichment above a stringent cutoff (log2 IP/input >0.25) (exploded section) among genes that are significantly differentially expressed upon ICRF-193 treatment (n=1,289/1,375 andn=349/1,375 respectively, depicted in blue). (d) Scatter plot relating expression changes (log2 scale) for genes significantly downregulated upon ICRF-193 treatment (ICRF/DMSO) (yaxis) to fold changes (log2 scale) during stem cell differentiation (TN/ES) (xaxis). Vertical red lines represent changes of 1.5-fold (linear) from ES to TN. (e) Scatter plot relating expression changes (log2 scale) for genes significantly upregulated upon ICRF-193 treatment (ICRF/DMSO) (yaxis) to fold changes (log2 scale) during stem cell differentiation (TN/ES) (xaxis). Vertical lines represent changes of 1.5-fold (linear) from ES to TN. Figure 5: Catalytic inhibition of TOP2 α misregulates target gene expression. ( a ) Volcano plot showing differentially expressed genes following ICRF-193 treatment as compared with DMSO in ESCs. The x axis shows fold changes in expression (log2 scale) and the y axis refers to the associated P -value (−log2 scale). The dotted red lines indicate the used cutoffs. Genes not expressed and expressed in DMSO treated samples are depicted in cyan and red respectively. ( b ) Scatter plot showing TOP2α enrichment at promoters ( y axis) of genes significantly misregulated (log2 scale) following ICRF-193 treatment ( x axis). ( c ) Pie chart representing the distribution of genes showing any TOP2α enrichment (log2 IP/input>0) or TOP2α enrichment above a stringent cutoff (log2 IP/input >0.25) (exploded section) among genes that are significantly differentially expressed upon ICRF-193 treatment ( n =1,289/1,375 and n =349/1,375 respectively, depicted in blue). ( d ) Scatter plot relating expression changes (log2 scale) for genes significantly downregulated upon ICRF-193 treatment (ICRF/DMSO) ( y axis) to fold changes (log2 scale) during stem cell differentiation (TN/ES) ( x axis). Vertical red lines represent changes of 1.5-fold (linear) from ES to TN. ( e ) Scatter plot relating expression changes (log2 scale) for genes significantly upregulated upon ICRF-193 treatment (ICRF/DMSO) ( y axis) to fold changes (log2 scale) during stem cell differentiation (TN/ES) ( x axis). Vertical lines represent changes of 1.5-fold (linear) from ES to TN. Full size image TOP2α controls pluripotency of ESCs Given our observations for a crucial role of TOP2α in regulating stem-cell transcriptome, we were next interested in investigating whether TOP2α inactivation impacts on molecular machinery underlying ES cell pluripotency and differentiation potential. Analysis of RNA-Seq data sets from TOP2α inhibited ESCs revealed a moderate but noticeable decrease in expression of a number of key pluripotency-related genes that were further validated in RT–qPCRs ( Fig. 6a ). These genes also showed a noticeable decrease in short-term TOP2α inhibition experiments, suggesting that they are the early responder genes in cells lacking TOP2α activity ( Supplementary Fig. S6a ). Furthermore, ICRF-193 misregulated genes include a number of genes that were recently described to define ESC state [39] ( Fig. 6b ). In addition, we find that TOP2α co-occupies a number of promoters with core stem-cell transcription factors such as KLF4, ESRRB and OCT4, but not NANOG ( Supplementary Fig. S6b ). Expression profiles of ICRF-193 misregulated genes in various mouse adult tissues revealed that these include genes expressed in all three lineages without any preference ( Supplementary Fig. S7 ), arguing for a function for TOP2α in defining expression potential of genes belonging to all lineages. In support of above observations for a role of TOP2α in regulating pluripotency, TOP2α inactivated ESCs, either with ICRF-193 or VP-16, fail to generate embryonic bodies and thus do not differentiate ( Fig. 6c ). Together these data clearly argue for a role of TOP2α in regulating pluripotency and differentiation potential of ESCs. 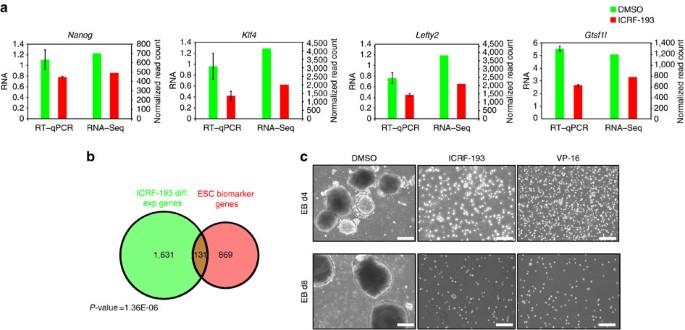Figure 6: TOP2αactivity is crucial for pluripotency and differentiation potential of mESCs. (a) Expression levels of selected pluripotency genes upon ICRF-193 treatment as measured by RNA-Seq as well as RT–qPCRs. mRNA levels were measured by RT–qPCR relative toRpl19and plotted on theyaxis. Error bars represent s.e.m. from two-independent biological replicates. Secondaryyaxis represents normalized read counts for the same genes from RNA-Seq experiments. (b) Venn diagram showing overlap between ICRF-193 misregulated genes with a set of genes described as biomarkers of the ESC state39.P-value of overlap was calculated using hypergeometric distribution with universal set as the total number of genes in the experiment (~20 K). (c) The morphology of embryoid bodies (EB) was monitored via phase contrast microscopy at four (EB d4) and eight days (EB d8) from the onset of differentiation. Microscopy pictures were taken at 10X magnification; scale bar, 200 μm. Figure 6: TOP2 α activity is crucial for pluripotency and differentiation potential of mESCs. ( a ) Expression levels of selected pluripotency genes upon ICRF-193 treatment as measured by RNA-Seq as well as RT–qPCRs. mRNA levels were measured by RT–qPCR relative to Rpl19 and plotted on the y axis. Error bars represent s.e.m. from two-independent biological replicates. Secondary y axis represents normalized read counts for the same genes from RNA-Seq experiments. ( b ) Venn diagram showing overlap between ICRF-193 misregulated genes with a set of genes described as biomarkers of the ESC state [39] . P -value of overlap was calculated using hypergeometric distribution with universal set as the total number of genes in the experiment (~20 K). ( c ) The morphology of embryoid bodies (EB) was monitored via phase contrast microscopy at four (EB d4) and eight days (EB d8) from the onset of differentiation. Microscopy pictures were taken at 10X magnification; scale bar, 200 μm. Full size image TOP2α is essential for genetic and epigenetic stability Having implicated TOP2α binding and catalytic activity in gene regulation, we next attempted to further validate expression changes observed in RNA-Seq experiments by single gene RT–qPCRs. The expression of analysed TOP2α target genes was consistently misregulated upon catalytic inhibition of TOP2α, while control genes remained unaffected ( Fig. 7a ). We next asked whether inhibition of TOP2α activity to resolve superhelical stress on DNA could lead to loss of DNA integrity at target promoters. Towards this we quantified levels of γH2AX, a marker of DNA double-strand breaks, by ChIP-qPCR in ICRF-193 or VP-16 treated samples. Interestingly, we observed a consistent enrichment of γH2AX at analysed TOP2α target promoters but not at control loci following such TOP2α inhibition ( Fig. 7b , Supplementary Fig. S8a ). VP-16 further led to accumulation of TOP2α at these sites ( Supplementary Fig. S8b ). Given high correlation of TOP2α with H3K4me2 ( Supplementary Fig. S1a ), we next investigated whether absence of TOP2α activity alters this chromatin mark. ChIP assay revealed a consistent decrease in H3K4me2 enrichment at TOP2α target promoters in TOP2α-inactivated cells ( Fig. 7c ) arguing that the lack of TOP2α activity not only results in loss of genomic integrity but also causes epigenetic changes at target promoters. 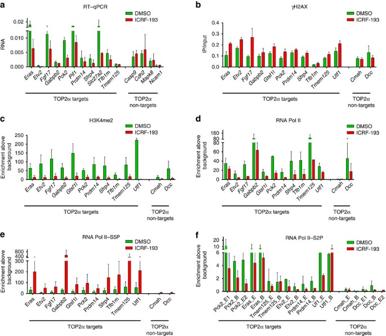Figure 7: TOP2αinhibition alters histone modification patterns and RNA Pol II kinetics. (a) mRNA levels were measured by RT–qPCR relative toRpl19(yaxis). Error bars indicate s.e.m. derived from two-independent biological replicates. (b) ChIP assay was performed using γH2AX-specific antibodies in DMSO and ICRF-193-treated cells followed by qPCR for promoters of genes shown in (a). Average enrichments, from three separate assays, are plotted on theyaxis as ratio of precipitated DNA (bound) to total input DNA. Error bars indicate s.e.m. (c) ChIP assay was carried out using H3K4me2-specific antibodies in DMSO and ICRF-193-treated cells and promoters of genes shown in (b) were amplified by qPCRs. This followed normalization to input and then an intergenic control region. Error bars reflect s.e.m. derived from two-independent biological replicates. (d) Following ChIP assay using an antibody detecting total RNA Pol II in DMSO- and ICRF-193-treated cells, the results were analysed and plotted as in (c). Error bars reflect s.e.m. derived from two-independent biological replicates. (e) Following ChIP assay using an antibody detecting the Ser5 phosphorylated form of RNA Pol II (RNA Pol II–S5P) in DMSO- and ICRF-193-treated cells, the results were analysed and plotted as in (c). Error bars reflect s.e.m. derived from two-independent biological replicates. (f) Following ChIP assay using an antibody detecting the Ser2 phosphorylated form of RNA Pol II (RNA Pol II-S2P) in DMSO- and ICRF-193-treated cells, the results were analysed and plotted as in (c), except that the primers used were designed for exons (E or E1) and exon intron boundaries (B) falling in the coding region and not promoters. One additional exon (E2), falling at the end of the coding region, was analysed for longer genes. Error bars reflect s.e.m. derived from two-independent biological replicates. Figure 7: TOP2 α inhibition alters histone modification patterns and RNA Pol II kinetics. ( a ) mRNA levels were measured by RT–qPCR relative to Rpl19 ( y axis). Error bars indicate s.e.m. derived from two-independent biological replicates. ( b ) ChIP assay was performed using γH2AX-specific antibodies in DMSO and ICRF-193-treated cells followed by qPCR for promoters of genes shown in ( a ). Average enrichments, from three separate assays, are plotted on the y axis as ratio of precipitated DNA (bound) to total input DNA. Error bars indicate s.e.m. ( c ) ChIP assay was carried out using H3K4me2-specific antibodies in DMSO and ICRF-193-treated cells and promoters of genes shown in ( b ) were amplified by qPCRs. This followed normalization to input and then an intergenic control region. Error bars reflect s.e.m. derived from two-independent biological replicates. ( d ) Following ChIP assay using an antibody detecting total RNA Pol II in DMSO- and ICRF-193-treated cells, the results were analysed and plotted as in ( c ). Error bars reflect s.e.m. derived from two-independent biological replicates. ( e ) Following ChIP assay using an antibody detecting the Ser5 phosphorylated form of RNA Pol II (RNA Pol II–S5P) in DMSO- and ICRF-193-treated cells, the results were analysed and plotted as in ( c ). Error bars reflect s.e.m. derived from two-independent biological replicates. ( f ) Following ChIP assay using an antibody detecting the Ser2 phosphorylated form of RNA Pol II (RNA Pol II-S2P) in DMSO- and ICRF-193-treated cells, the results were analysed and plotted as in ( c ), except that the primers used were designed for exons (E or E1) and exon intron boundaries (B) falling in the coding region and not promoters. One additional exon (E2), falling at the end of the coding region, was analysed for longer genes. Error bars reflect s.e.m. derived from two-independent biological replicates. Full size image We next investigated whether TOP2α activity affects the recruitment, initiation and/or elongation of RNA Polymerase II at the target genes. ChIP assay revealed that ICRF-193 treatment led to a decrease in the total Pol II levels at these promoters ( Fig. 7d ). Moreover, such TOP2α inactivation also led to increased enrichment of the initiating form of RNA Pol II (RNA Pol II–S5P) at these promoters ( Fig. 7e ) and reduction in the elongating form of RNA Pol II (RNA Pol II–S2P) at gene bodies ( Fig. 7f ). These observations suggest that ICRF-193-mediated inhibition of TOP2α activity not only reduces further recruitment of RNA Pol II, but also prevents the release of the initiating form at the target promoters. Topoisomerases represent the second most abundant chromatin protein in eukaryotes after histones and ensure DNA integrity during fundamental biological processes [4] , [5] , [6] . Unlike its isozyme TOP2β that is robustly expressed upon terminal differentiation, TOP2α is highly abundant in rapidly dividing cells such as pluripotent ES cells and is indispensable [8] , [15] , [16] , [17] , [18] . Furthermore, targeted disruption of Top2a gene caused embryonic lethality at 4 or 8-cell stage, suggesting its essential role during early mouse development [12] . Driven by our recent findings for a gene regulatory role of TOP2β during neuronal differentiation, we were tempted to address whether TOP2α may also contribute to transcriptional regulation, especially in the context of maintaining stem-cell properties. Furthermore, despite exhibiting similar enzymatic activity in vitro , we still lack information about similarities and differences between the genomic targets and function of the two Topo II isozymes. Here we show that TOP2α and TOP2β expression are characteristics of dividing, pluripotent and postmitotic, differentiated cells, respectively. We discovered an unexpected universal recruitment of TOP2α to promoters of a large number of genes in ESCs. These promoters are defined by distinct histone modifications and are largely transcribed. However, a small number of TOP2α target genes that are not expressed are marked with bivalent chromatin, a state defined by the co-occurrence of H3K4 and H3K27 methylation. Such coexistence of active and repressive marks is thought to mark developmental genes in ESCs poised for later activation upon differentiation [40] . Interestingly, a significant number of these TOP2α target genes resolve the bivalent chromatin state upon differentiation into neurons that accompanies their expression and binding by TOP2β. We therefore speculate that TOP2α binding at bivalently marked developmental genes in stem cells contributes to their immediate activation upon differentiation. TOP2α catalytic activity might keep their promoter chromatin in an accessible state, thereby facilitating targeting by development-specific transcription factors that become expressed upon differentiation. Similar priming by TOP2α in ESCs was observed for large length target genes (>250 kb) that were subsequently bound by TOP2β and expressed upon differentiation. It is possible that long length makes these genes indispensably dependent on topoisomerase II activity and therefore, it is absolutely required for them to be acted upon by TOP2α in stem cells to ensure their proper transcription upon differentiation that accompanies functional takeover by TOP2β. Indeed, we find that these genes rely on TOP2α activity for ensuring a more accessible chromatin state in stem cells. Together, these findings suggest a role for TOP2α in priming development-specific genes for activation and TOP2β binding upon differentiation. H3K4 methylation at promoters associates with active transcription and several enzymes methylate and demethylate this residue in higher eukaryotes [41] , [42] . A number of proteins are increasingly being discovered that recognize H3K4 modifications, suggesting that these modifications primarily serves to recruit a multitude of proteins onto chromatin and repel others [43] , [44] , [45] . Such recruitment of chromatin-modulating enzymes would result in structural constraints that may require topoisomerase activity to maintain genomic integrity and ensure proper gene regulation. We find that absence of TOP2α activity accompanies changes in H3K4me2 enrichments at target promoters, suggesting a link between this modification and function of TOP2α. TOP2α targets are largely transcribed in ESCs and enriched for housekeeping function as well as pluripotency regulation such as cytokine signalling pathways. It is well established that small molecules such as the interleukin 6 class cytokine LIF are critical regulators of ESC pluripotency [31] , [46] . Our transcriptome profiling in ESCs lacking TOP2α activity revealed significant changes in gene expression program. Importantly, majority of genes significantly misregulated upon ICRF-193 treatment were TOP2α bound, suggesting that its enzymatic activity directly contributes to their transcriptional regulation. Among these, downregulated genes were enriched in GO processes for metabolism, signalling, proliferation and transcriptional regulation, whereas upregulated genes consist of cell-fate commitment, development and neurogenesis genes. Interesting to note that even if a large fraction of TOP2α targets are housekeeping genes, only a small number of these were affected upon inhibition of TOP2α activity. These housekeeping genes are very highly expressed compared with other ICRF-193 misregulated genes. This might explain the inability to detect a strong effect on their transcription, especially under the low dose and short duration ICRF-193 treatment conditions we employed to minimize potential secondary effects and capture the most responsive genes. Furthermore, given critical importance of housekeeping genes in maintaining cellular homeostasis, it is also possible that organisms have evolved mechanisms to tightly balance their expression under perturbed conditions. Interestingly, a significant fraction of genes misregulated upon ICRF-193 treatment show similar changes in expression during stem-cell differentiation into neurons that accompanies a natural depletion of TOP2α. These misregulated genes included those linked to the maintenance of stem-cell state [39] and consisted of classical pluripotency genes that were downregulated. Moreover, TOP2α and core stem-cell transcription factors such as KLF4, ESRRB and OCT4 co-occupy a number of genes, further suggesting contribution of TOP2α in conferring stem-cell identity. The ICRF-193 misregulated genes do not show preference for expression in any particular lineage, supporting the known broad developmental potential of ESCs and arguing for a function for TOP2α in defining expression potential of genes belonging to all lineages. Together with our observations that these TOP2α inhibited cells show lack of differentiation ability, we conclude a critical role of TOP2α in defining stem-cell pluripotency and differentiation potential. However, even though we provide ample evidence that loss of pluripotency underlies defects following TOP2α inhibition, it is not possible to absolutely tease apart the effects resulting from influence on proliferation than authentic pluripotency, especially as these two aspects are critically linked to each other in defining stem-cell state. Large-scale functional experiments need to be performed to generate a comprehensive view of how TOP2α and its target genes are connected to the complex network that regulates self-renewal and pluripotency of ESCs [47] , [48] , [49] , [50] . Given that TOP2α target sites display defined histone modification patterns, we speculated for a crosstalk between TOP2α binding and the epigenetic state of target promoters. Indeed, absence of TOP2α activity accompanies alterations in histone modifications, as exemplified by changes in γH2AX and H3K4me2 enrichments. As a consequence, it is possible that different gene regulatory complexes are recruited at the target promoters that mediate altered transcriptional response [51] , [52] , [53] . Future work will establish whether changes in chromatin composition is a cause or consequence of transcriptional aberrations that follow TOP2α inhibition. Our findings in cells lacking TOP2α activity shows that TOP2α may mediate RNA Pol II recruitment and promote the release of the initiating form for active transcription. As we detect TOP2α at certain promoters in the absence of RNA Pol II, it is possible that TOP2α is recruited before actual transcriptional activation and may have a role in recruiting and promoting RNA Pol II function at transcriptionally active loci. These findings are in agreement with observation made in yeast [54] , [55] and provide fundamental insights into the mechanism how these enzymes may constitute an important layer of the gene regulatory network. Taken together, our findings provide novel insights into genomic localization and gene regulatory function of TOP2α in ESCs as well as its relationship and differences with TOP2β. Our results suggest a model for a dual function of TOP2α in ESCs where it not only directly contributes to transcriptional regulation of a specific set of genes but also primes developmental genes for subsequent activation upon differentiation ( Fig. 8 ). Our findings provoke for a major paradigm shift in the concepts of how labour is divided between the two topo II isoforms and how these enzymes are involved in gene regulation. It is very exciting to uncover how these enzymes, classically known to support chromosomal integrity by resolving torsional stress, participate in gene regulatory networks that is not only important for maintenance of cell-identity but also for developmental decisions. Future work should aim to unravel how the collaborative partnership between the two topo II isoforms contributes to transcriptional reprogramming underlying tri-lineage differentiation during embryonic development. 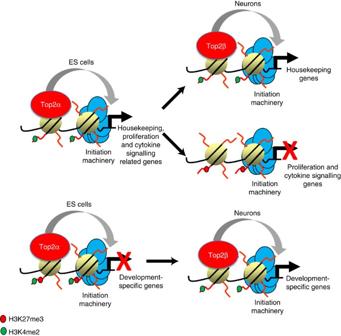Figure 8: Model for a dual role of TOP2αin ESCs. TOP2α contributes to the transcriptome regulation in ESCs especially for genes involved in housekeeping function as well as proliferation and cytokine signalling (upper panel). Following differentiation to neurons, housekeeping genes continue to express and become bound by TOP2β, while proliferation and cytokine signaling genes are shut down. In addition, TOP2α has a priming function at development-specific genes, which are pre-bound by TOP2α but not transcribed in ESCs and upon differentiation get expressed and occupied by TOP2β (lower panel). Figure 8: Model for a dual role of TOP2 α in ESCs. TOP2α contributes to the transcriptome regulation in ESCs especially for genes involved in housekeeping function as well as proliferation and cytokine signalling (upper panel). Following differentiation to neurons, housekeeping genes continue to express and become bound by TOP2β, while proliferation and cytokine signaling genes are shut down. In addition, TOP2α has a priming function at development-specific genes, which are pre-bound by TOP2α but not transcribed in ESCs and upon differentiation get expressed and occupied by TOP2β (lower panel). Full size image Cell culture Wild-type mouse ESCs derived from blastocysts (3.5 PC) of pregnant females of mixed 129-C57Bl/6 background (called 159.2) were cultured at 37 °C, 7% CO 2 and 88% relative air humidity in 8 ml ES medium (DMEM supplemented with 10% fetal calf serum, 2 mM L -glutamine and LIF on feeders (inactivated MEFs). For further experiments, feeders were removed by splitting mESCs every 2 days on tissue-culture dishes coated with 0.2% gelatin with daily media change. Experiments were performed at feeder-free five state. Catalytic inhibition of TOP2 α Feeder-free ESCs were seeded at a density of 3.3 × 10 6 cells in 10 cm dishes and cells were treated after 32 h for 16 h with 500 nM ICRF-193 (or 500 nM VP-16) (Sigma) or DMSO as a control before proceeding for further experiments. Cell cycle analysis ESCs were pulse treated with 10 μM BrdU for 2 h. Cells were trypsinized, fixed for 10 min with 4% paraformaldehyde, washed with PBS and permeabilized overnight at −20 °C using 80% cold MeOH in PBS. Cells were washed twice with PBS and staining was performed using BD Pharmingen BrdU Flow Kits according to manufactures instructions. DNA counterstain was performed using 25 μg of DAPI along with RNase (0.1 mg ml −1 final concentration) digest for 30 min. Samples were subsequently measured using the BD LSRFortessa Cell Analyser with BD FACSDiva software and plots were generated using FlowJo. ChIP ES cells were crosslinked in medium containing 1% formaldehyde for 10 min at room temperature, scraped off and rinsed with 10 ml 1 × PBS. Pellets were resuspended in 10 ml buffer 1 (10 mM Tris (pH 8.0), 10 mM EDTA, 0.5 mM EGTA, 0.25% Triton X-100) and once in 10 ml buffer 2 (10 mM Tris (pH 8.0), 1 mM EDTA, 0.5 mM EGTA, 200 mM NaCl). Next, cells were lysed in 900 μl lysis buffer (50 mM HEPES/KOH (pH 7.5), 500 mM NaCl, 1 mM EDTA, 1% Triton X-100, 0.1% DOC, 0.1% SDS, protease inhibitors) and sonicated using Bioruptor plus (Diagenode). Precleared chromatin (60 μg) was incubated overnight at 4 °C with respective antibodies (TOP2α: sc5346x (Santa Cruz), γH2Ax: 05-636 (Millipore), anti-TOP2β: H286 (Santa Cruz), RNA Pol II: N-20 (Santa Cruz), H3K4me2: 07030 (Millipore), H3K27me3: 07-449 (Millipore), RNA Pol II: sc899 (Santa Crutz), RNA Pol II Ser2: ab5095 (abcam) and RNA Pol II Ser5: ab5131 (abcam)) and then incubated for 3 h at 4 °C with 40 μl protein A-Sepharose beads preblocked with tRNA and BSA. Beads were washed twice with 1 ml lysis buffer and once with 1 ml DOC buffer (10 mM Tris (pH 8.0), 0.25 M LiCl, 0.5% NP-40, 0.5% deoxycholate, 1 mM EDTA), and bound chromatin was eluted in 1% SDS/0.1 M NaHCO 3 . This followed treatment with RNase A (0.2 mg ml −1 ) for 30 min at 37 °C and then with proteinase K (50 μg ml −1 ) for 2.5 h at 55 °C. The crosslinking was reversed at 65 °C overnight with gentle shaking. DNA was purified by phenol–chloroform extraction followed by ethanol precipitation and recovered in 40 μl TE buffer. Real-time PCR on ChIP (1:40) or input (1:100) DNA was performed using SYBR Green chemistry (ABI). ChIP-chip or ChIP-seq was performed using this material. FAIRE ES cells treated with either DMSO or 500 nM ICRF-193 were crosslinked as described for ChIP assay above. Cells were collected by scraping in cold PBS and resuspended in 3 ml of buffer L1 (50 mM HEPES/KOH, pH 7.5, 140 mM NaCl, 1 mM EDTA pH 8.0, 10% glycerol, 5% NP-40, 0.25% Triton X-100) and incubated for 10 min at 4 °C. This was followed by centrifugation for 5 min at 4 °C at 1,300 g . The pellet was then resuspended in 3 ml of buffer L2 (200 mM NaCl, 1 mM EDTA pH 8.0, 0.5 mM EGTA pH 8.0, 10 mM Tris pH 8.0) and incubated for 10 min at room temperature, followed by centrifugation for 5 min at 4 °C at 1,300 g . The pellet was then resuspended in 600 μl buffer L3 (1 mM EDTA pH 8.0, 0.5 mM EGTA pH 8.0, 10 mM Tris pH 8.0, 100 mM NaCl, 0.1% Na-deoxycholate, 0.17 mM N -lauroyl sarcosine) containing protease inhibitors and incubated at 4 °C for 3 h. Samples were then sonicated using Bioruptor plus (Diagenode) and cellular debris was cleared by spinning at 14,000 g for 10 min at 4 °C. DNA was isolated by adding an equal volume of phenol:chloroform:isoamylalcohol (25:24:1), vortexing and spinning at 12,000 g for 5 min at room temperature. The aqueous phase was isolated and a second round of phenol:chloroform:isoamylalcohol purification was performed. Following collection of aqueous phase, chloroform:isoamylalcohol (24:1) was added, vortexed and spun at 12,000 g for 5 min at room temperature. The aqueous phase was then collected and DNA was ethanol precipitated and recovered in 40 μl TE buffer. This recovered material was then re-cleaned with phenol followed by chloroform:isoamylalcohol (24:1) and subsequently ethanol precipitated. Next, DNA was recovered in 40 μl TE buffer. For deriving input DNA control, RNase and proteinase K digestion, reverse crosslinking and purification of 10% input material was performed as described for ChIP samples. Real-time RT–PCR RNA was isolated using SurePrep TrueTotal RNA Purification Kit (Fisher Scientific) and subsequently used for cDNA synthesis applying First Strand cDNA Synthesis Kit (Fermentas). Expression levels of genes were measured using SYBR Green chemistry (ABI). Primer sequences are provided as Supplementary Table S6 . ChIP-chip data analysis NimbleGen array intensity files were read, and log2 enrichments (log2 bound/input ratios) for each individual probe were calculated using the R package Ringo [56] . To remove dye artifacts, both arrays were loess-normalized using the ‘normalizeWithinArrays’ function and were also normalized using ‘normalizeBetweenArrays’ function from the limma package [57] . To calculate log2 enrichments for different genomic regions (promoters, exons, introns and intergenic), log2 enrichments of all probes that mapped to a particular region were averaged. RNA-Seq analysis RNA-Seq libraries were generated according to Illumina’s instructions using oligo-dT primers. Reads were aligned to mouse genome (mm9) using TopHat [58] with default parameters. The aligned reads were then provided as an input to HTSeq_count utility from HTSeq package. The raw read count files obtained from HTSeq-count were then processed for differential expression using DESeq package [59] . The raw read counts were normalized for library size differences using estimate size factors function from DESeq package. Tissue-specific data sets were obtained from Gene Expression Omnibus with following GEO accession numbers: GSM929705 , GSM929717 , GSM929709 , GSM929708 , GSM929707 , GSM929706 , GSM929711 , GSM929721 , GSM652441 , GSE33922 , GSE33922 , GSE33922 and GSE38805 . The data were processed as mentioned above with additional VSD normalization using DESeq package [59] . FAIRE-Seq analysis The FAIRE libraries processed for Illumina sequencing were prepared according to Illumina’s instructions (Catalogue number IP-102-1001). Reads were aligned to mouse genome (mm9) using Bowtie [60] with default parameters. Aligned reads of all replicates from DMSO- and ICRF-193-treated cells were merged together to generate a single input fastq file. This merged fastq file was given as input to Fseq package [61] using default options to identify all potential peaks from combined samples. The peaks reported by FSeq were again filtered based on enrichment and only peaks with enrichment above input were considered for investigating accessibility differences in long silent genes between DMSO- and ICRF-193-treated samples. Immunoprecipitation enrichment of genomic regions/peaks was calculated as E =log 2 (( n FG / N FG × min( N FG , N BG )+p)/( n BG / N BG × min( N FG , N BG )+ p )), where n FG and n BG are reads aligned in foreground and background (input chromatin) alignments in a particular genomic region, N FG and N BG are the total number of aligned reads in foreground and background samples, and p is a pseudocount constant used to regularize enrichments with low counts dominated by sampling noise. Accession codes : The ChIP-chip, RNA-Seq and FAIRE-Seq data has been deposited in Gene Expression Omnibus under accession code GSE46070 . How to cite this article: Thakurela, S. et al. Gene regulation and priming by topoisomerase IIα in embryonic stem cells. Nat. Commun. 4:2478 doi: 10.1038/ncomms3478 (2013).